Tandem C–H oxidation/cyclization/rearrangement and its application to asymmetric syntheses of (−)-brussonol and (−)-przewalskineE Natural products are a vital source of lead compounds in drug discovery. Development of efficient tandem reactions to build useful compounds and apply them to the synthesis of natural products is not only a significant challenge but also an important goal for chemists. Here we describe a tandem C–H oxidation/cyclization/rearrangement of isochroman-derived allylic silylethers, promoted by DDQ and InCl 3 . This method allows the efficient construction of tricyclic benzoxa[3.2.1]octanes with a wide substrate scope. We employ this tandem reaction to achieve the asymmetric total syntheses of (−)-brussonol and (−)-przewalskine E . The strained tricyclic benzoxa[3.2.1]octane skeleton exists in numerous bioactive and pharmaceutical molecules such as przewalskone [1] and brussonol [2] , and it is a useful building block in organic synthesis such as for producing platensimycin [3] ( Fig. 1a ). In recent decades, the significant biological activity and potential pharmaceutical value of molecules with this skeleton have driven chemists to devise several methods for constructing it ( Fig. 1b ) [3] , [4] , [5] , [6] , [7] , [8] , [9] , [10] , [11] , [12] , [13] , [14] . Nevertheless, more efficient and practical methods are needed. 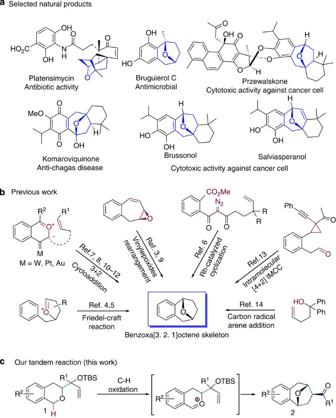Figure 1: Representative natural products containing benzoxa[3.2.1]octane skeleton and approaches to it. (a) Selected bioactive natural products having benzoxa[3.2.1]octane skeleton. (b) Previous methods for construction of benzoxa[3.2.1]octane skeleton. (c) Our synthetic proposal via a tandem C–H oxidation/cyclization/rearrangement reaction. Figure 1: Representative natural products containing benzoxa[3.2.1]octane skeleton and approaches to it. ( a ) Selected bioactive natural products having benzoxa[3.2.1]octane skeleton. ( b ) Previous methods for construction of benzoxa[3.2.1]octane skeleton. ( c ) Our synthetic proposal via a tandem C–H oxidation/cyclization/rearrangement reaction. Full size image One possible approach is the C–C bond formation via direct (sp 3 ) α-C–H bond functionalization, which is increasingly being used to synthesize complex N- or O-containing molecules [15] , [16] , [17] , [18] . While several reactions have been described to achieve C–C formation at the α-position in amines, only a handful of reactions have been reported for C–C formation in ethers [19] , [20] , [21] , [22] , [23] , [24] , [25] , [26] , [27] , [28] , [29] . In connection with our long-standing interest in α-C–H bond functionalization of ethers [30] , [31] and in carbon–carbon rearrangement of allylic alcohol/silylether [32] , [33] , [34] , we speculated that it might be possible to construct the benzoxa[3.2.1]octane unit via a tandem reaction that is initiated by benzylic C–H oxidation of an isochroman-derived allylic silylether and triggered by C–C bond rearrangement. Here we use 2,3-dichloro-5,6-dicyanobenzoquinone (DDQ) and InCl 3 to promote tandem C–H oxidation/cyclization/rearrangement of isochroman-derived allylic silylether. We then apply this efficient tandem reaction to asymmetric syntheses of the bioactive natural products (−)-brussonol and (−)-przewalskine E . Reaction optimization We began our efforts to generate the benzoxa[3.2.1]octane unit using the model substrate 1a, prepared as a single diastereoisomer in a general procedure (see Supplementary Methods 1 and Supplementary Data 1 and 4 ). Initial experiment with the common oxidant DDQ (2.0 equiv.) as the sole promoter failed to give the desired product and resulted in fully recovery of 1a ( Table 1 , entry 1). Next we tried combinations of DDQ (1.2 equiv.) and Lewis acids in the presence of 4-Å molecular sieve. Using FeCl 3 or SnCl 4 led to the decomposition of 1a (entries 2 and 3), whereas using SnBr 4 led to the consumption of 1 a in 8 h and the desired product 2a in 33% yield (entry 4). Cu(OTf) 2 and LiClO 4 also promoted this transformation, albeit in lower yield (entries 5 and 6). When 1.0 equiv. InCl 3 was used, 2a was obtained in 36% yield after 24 h and 15% of 1a was recovered (entry 7). Increasing the load of DDQ to 2.0 equiv. gave higher yield (56%) in shorter time (4 h). Interestingly, decreasing the load of InCl 3 to 0.1 equiv. further increased the yield of 2a to 69% (entry 9). The molecular sieve was essential to this reaction, since omitting it led to only 30% yield (entry 10). With InCl 3 as the catalyst, a side reaction in which 1a was partially desilylated to give free allylic alcohol was always observed. To inhibit this, we screened several weakly basic additives (entries 11–14). We were pleased to find that using 2,6-dibromopyridine (DBP, 5.0 equiv.) significantly improved yield to 81% (entry 14). In addition, the reaction was also carried out in some other solvents (C 2 H 4 Cl 2 , CH 3 NO 2 , CH 3 CN, toluene, tetrahydrofuran (THF)) and oxidants (TEMPO, benzoquinone), but results were not better than with CH 2 Cl 2 and DDQ. Therefore, the optimal conditions were defined to be DDQ (2.0 equiv. ), InCl 3 (0.1 equiv. ), DBP (5.0 equiv.) and 4-Å molecular sieve in CH 2 Cl 2 (entry 14, see Supplementary Methods 2 ). Table 1 Conditions optimization*. Full size table Substrate scope Using these optimal reaction conditions, we tested the substrate scope of this transformation extensively ( Fig. 2 ), starting with the allylic substituents at R 1 . Substrates 1b and 1c with n -butyl and i -propyl groups at this position reacted well and gave the desired products 2b and 2c in respective yields of 80 and 83%. Benzyl-substituted 1d also afforded the desired product 2d in good 72% yield. In contrast, substrates with more electron-rich groups at R 1 gave only medium to good yields. For example, substrates 1e and 1f with phenyl and vinyl substituents gave the corresponding products 2e and 2f in respective yields of 74 and 63% yield. The substrate 1g with an acetylenyl substituent generated the product 2g in a lower yield of 23%. Using substrate 1h with a methyl substitution at the ally C=C led to smooth production of 2h with a quaternary stereocenter in 83% yield. The product’s relative configuration was confirmed by X-ray diffraction analysis. Next, the substituent effects on the aromatic ring of the isochroman moiety were investigated—compounds 1i and 1j fully substituted with MeO or Me reacted well, giving products 2i and 2j in respective yields of 83 and 87%. These relatively high yields may mean that the electron-donating methoxyl group stabilizes the benzylic oxonium carbocation in the transition state in Fig. 1c better than hydrogen does. Compound 1k with a bromo substituent at the 7th position in the isochroman moiety led to the desired product 2k in 63% yield, extending the flexibility of our approach for further derivatization. 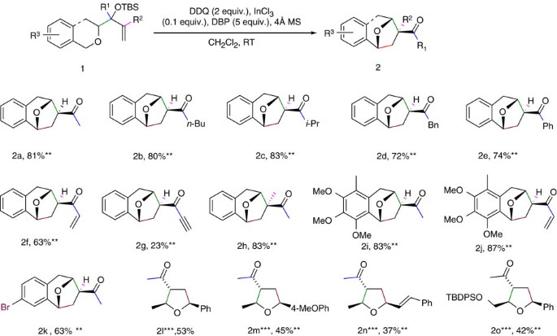Figure 2: Reaction scope*. *All reactions unless notified were performed in experimental section procedure on a 0.1–1.5 mmol substrate scale in CH2Cl2(0.1 mmol ml−1), 0.1 equiv. InCl3, 4 Å MS (50 mg per 0.1 mmol), 2.0 equiv. DDQ, 5.0 equiv. DBP at RT. Relative configuration of the products were assigned based on X-ray structure of2hand2j(CCDC 1000811, CCDC 1000827, SeeSupplementary Data 2 and 3for more details). **Isolated yields. ***1.1 equiv. DDQ was used. Figure 2: Reaction scope*. *All reactions unless notified were performed in experimental section procedure on a 0.1–1.5 mmol substrate scale in CH 2 Cl 2 (0.1 mmol ml −1 ), 0.1 equiv. InCl 3 , 4 Å MS (50 mg per 0.1 mmol), 2.0 equiv. DDQ, 5.0 equiv. DBP at RT. Relative configuration of the products were assigned based on X-ray structure of 2h and 2j (CCDC 1000811, CCDC 1000827, See Supplementary Data 2 and 3 for more details). **Isolated yields. ***1.1 equiv. DDQ was used. Full size image We also expanded the substrate scope to acyclic systems to allow the synthesis of multi-substituted THF derivatives, which exist in numerous bioactive and pharmaceutical molecules [35] , [36] , [37] . Four representative allylic siylethers 1l – 1o with terminal benzylic or allylic ethers as the reaction trigger generated the corresponding products 2l – 2o in 37–53% yields under the same optimal conditions. Notably, the reaction was triggered efficiently by either benzylic ethers ( 1l , 1m , 1o ) or cinnamylic ethers. ( 1n ) When a TBDPS ethylene ether was created in 1o to compete with benzyl ether during the expected reaction, only the benzyl ether underwent reaction, affording the product 2o in 42% yield. Under the same optimal conditions, yields were generally lower with acyclic substrates than with cyclic ones, which may be due to hyperoxidation of THF products that produced furan-type by-products ( Supplementary Methods 2.2 ). Asymmetric syntheses of (−)-brussonol and (−)-przewalskine E To further demonstrate the utility of this novel method for synthesizing polycyclic molecules, we applied it to the total synthesis of two important bioactive natural products—tetracyclic (−)-przewalskine E ( 3a) and (−)-brussonol ( 3b ) [2] , [38] , [39] , [40] . Two diastereoselective routes to 3b have been reported by Sarpong [41] and Jennings [42] , while its asymmetric synthesis has been achieved by Majetich [43] . We are unaware of reports of the synthesis of 3a . In our retrosynthetic analysis ( Fig. 3 ), we hypothesized that we could generate 3a from 3b via biomimetic oxidation, and that 3b could be obtained from ketone intermediate 3c . We planned to construct rings C and D in 3c by applying our novel method to the tricyclic allylic siylether 3d, which could be obtained from achiral allylic alcohol 3e via a challenging tandem Sharpless asymmetric epoxidation/epoxy opening. The precursor 3e could be prepared from the simple starting material 3f [44] in a few short steps. 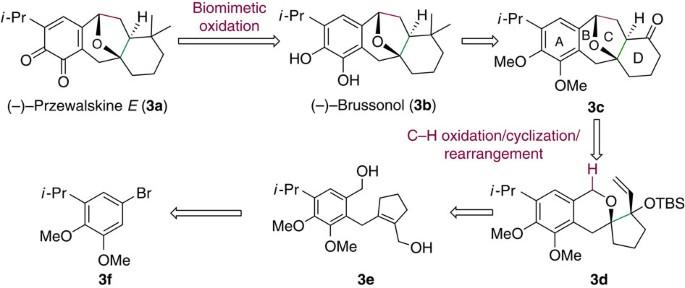Figure 3: Retrosynthetic analysis of3a,b. The current method was used to construct the core framework. Figure 3: Retrosynthetic analysis of 3a,b . The current method was used to construct the core framework. Full size image On the basis of this strategy, we started our synthesis by preparing allylic alcohol 3e from bromide 3f ( Fig. 4 ), which was formalized and protected as a 1,3-dioxane 3g to survive subsequent metallization [45] , [46] . Deprotonation of 3g with n -BuLi followed by quenching with formaldehyde and finally bromination of the resulting hydroxyl group with Ph 3 P/CBr 4 gave benzyl bromide 3h in 41% yield over two steps. Coupling bromide 3h with vinyl triflate 3i [47] and then removing the 1,3-dioxane protecting group in aqueous HCl afforded aldehyde 3j in 69% yield over two steps. Excess diisobutylaluminum hydride (DIBAL-H) was used to reduce 3j in a single step to diol 3e in 93% yield. Then we investigated the key tandem Sharpless asymmetric epoxidation/epoxy opening of 3e . The expected tricyclic species 3k was obtained in 90% yield and 83% ee in the presence of classic Sharpless catalyst (1.5 equiv.) at −50 °C. While this enantioselectivity is not ideal, it appears to be a rare example of successful tetra -substituted olefin epoxidation [48] . Selective oxidation of the primary hydroxyl of 3k followed by methylenenation afforded the desired tertiary allylic alcohol 3l , which was protected to give the precursor 3d . Fortunately, our optimal conditions of oxidative cyclization/ring enlargement gave the expected tetracyclic skeleton 3c in high yield (81%) and excellent stereoselectivity, no other isomer was detected. 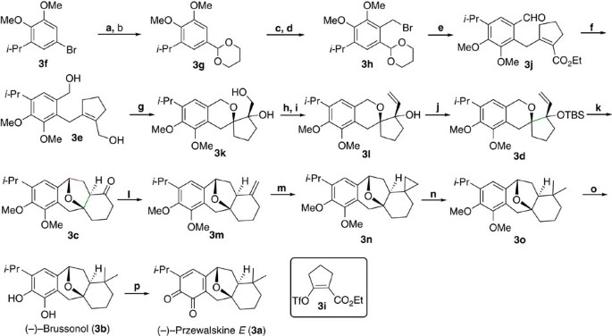Figure 4: Asymmetric total synthesis of (−)-przewalskineE(3a) and (−)-brussonol (3b). Reagent and conditions: (a)n-BuLi, Et2O, −78 °C, then DMF; (b) 1,3-propanediol, CH(OEt)3, (n-Bu)4N+Br3-, 65 °C; 77% (2 steps); (c)n-BuLi, Hexane/Et2O, RT, then CH2O in THF, −78 °C; (d) Ph3P, CBr4, CH2Cl2, 0 °C, 41% (2 steps); (e) (i) Zn, THF, 0 °C to RT, then Pd(Ph3P)2Cl2,3iin DMF, 90 °C; (ii) 4 mol l−1HCl, THF/H2O (4:1), 69% (2 steps); (f) DIBAL-H, CH2Cl2, −78 °C to RT, 93%; (g) (−)-DET, Ti(i-PrO)4,t-BuO2H, −25 °C to −50 °C, CH2Cl2, 90% yield, 83% ee; (h) DMSO, DIPEA, SO3·Py, CH2Cl2;(i) Ph3PCH3Br,t-BuOK, Tol, 72% (2 steps); (j) TBSOTf, Et3N, CH2Cl2, 0 °C to 40 °C, 98%; (k) 4 Å MS, 2,6-DBP, InCl3, DDQ, CH2Cl2, RT, 82%; (l) Ph3PCH3Br,t-BuOK, Toluene, 88%; (m) Et2Zn, CH2I2, Tol., 58%; (n) Pt2O, H2(1 atm), AcOH, 65 °C, 89%; (o) EtSH, NaH, DMF, 150 °C, 76%; (p) Ag2O, Et2O, RT, 71%. DIPEA,N,N-diisopropylethylamine. Figure 4: Asymmetric total synthesis of (−)-przewalskine E (3a) and (−)-brussonol (3b). Reagent and conditions: ( a ) n -BuLi, Et 2 O, −78 °C, then DMF; ( b ) 1,3-propanediol, CH(OEt) 3 , ( n -Bu) 4 N + Br 3 - , 65 °C; 77% (2 steps); ( c ) n -BuLi, Hexane/Et 2 O, RT, then CH 2 O in THF, −78 °C; ( d ) Ph 3 P, CBr 4 , CH 2 Cl 2 , 0 °C, 41% (2 steps); ( e ) (i) Zn, THF, 0 °C to RT, then Pd(Ph 3 P) 2 Cl 2 , 3i in DMF, 90 °C; (ii) 4 mol l −1 HCl, THF/H 2 O (4:1), 69% (2 steps); ( f ) DIBAL-H, CH 2 Cl 2 , −78 °C to RT, 93%; ( g ) (−)-DET, Ti( i- PrO) 4 , t -BuO 2 H, −25 °C to −50 °C, CH 2 Cl 2 , 90% yield, 83% ee; ( h ) DMSO, DIPEA, SO 3 ·Py, CH 2 Cl 2 ;( i ) Ph 3 PCH 3 Br, t -BuOK, Tol, 72% (2 steps); ( j ) TBSOTf, Et 3 N, CH 2 Cl 2 , 0 °C to 40 °C, 98%; ( k ) 4 Å MS, 2,6-DBP, InCl 3 , DDQ, CH 2 Cl 2 , RT, 82%; ( l ) Ph 3 PCH 3 Br, t -BuOK, Toluene, 88%; ( m ) Et 2 Zn, CH 2 I 2 , Tol., 58%; ( n ) Pt 2 O, H 2 (1 atm), AcOH, 65 °C, 89%; ( o ) EtSH, NaH, DMF, 150 °C, 76%; ( p ) Ag 2 O, Et 2 O, RT, 71%. DIPEA, N , N -diisopropylethylamine. Full size image At this stage, only the installation of a gem-dimethyl group remained to complete the synthesis of 3b . Initial attemps to transform the carbonyl in ketone 3c directly into gem-dimethyl using TiMe 2 Cl 2 reagent [49] gave the desired product 3o in low yield. Therefore, we adopted a three-step protocol involving Wittig reaction, cyclopropanation and reduction. Treating 3c with Ph 3 PCH 3 Br/ t -BuOK followed by Simmons–Smith cyclopropanation of the resulting exo-cyclic olefin gave the cyclopropane compound 3n , which was hydrogenated with H 2 (1 atm)/PtO 2 to afford the desired 3o in 45% yield over three steps [50] . Demethylating 3o using with EtSNa/DMF provided natural product 3b in 76% yield, and the spectral data were identical to those reported by Sarpong [41] ( Supplementary Tables 1 and 2 ). We screened various oxidants for the biomimetic oxidation of 3b to 3a ; Ag 2 O proved to be the best, affording the natural product 3a in 71% yield. Its spectral data were identical to those reported by Zhao [40] ( Supplementary Tables 3 and 4 ). The tandem C–H oxidation/cyclization/rearrangement of isochroman-derived allylic silylether described here shows good chemo- and stereoselectivity as well as good product yield. We demonstrated the usefulness of this approach by using it to achieve the asymmetric total syntheses of (−)-brussonol and (−)-przewalskine E . We expect that this approach will find additional applications in organic synthesis. This approach involves simpler initiation and substrate preparation as well as milder reaction conditions than a similar acetal rearrangement under acidic conditions via alkoxy release reported by Overman’s group [51] , [52] , [53] , [54] , [55] , [56] , [57] , [58] . Notably, we nearly always obtained the desired product with a benzoxa[3.2.1]octane framework as a single diastereomer ( Fig. 2 ). In term of the mechanism of this transformation, there are two possible pathways whereby intermediate B may react with a benzylic oxocarbenium cation under oxidative conditions ( Fig. 5 ). One is a tandem cyclization/semipinacol rearrangement to give E (pathway a) and the other is a tandem [3,3]-Cope rearrangement/aldol reaction (pathway b) [52] . Our results suggest that pathway b is more likely, since we did not obtain products with a benzoxa[3.3.1] skeleton when we used substrates 1e , 1f , 1g or 1j , all of which should preferentially undergo migration of an electron-rich R 1 group when a semipinacol rearrangement process is involved. In addition, both substrates 1h and 1h′ , which are epimers at the allylic position, gave a single diastereomeric product. Whether pathway b is the true one under our optimal conditions needs to be confirmed. 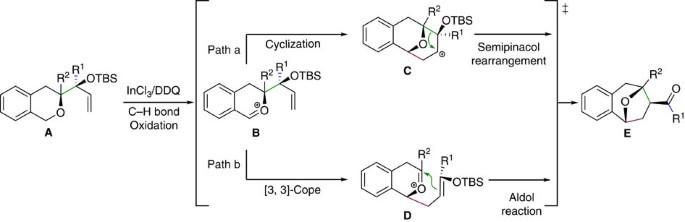Figure 5: Proposed mechanism. (a) Tandem C–H bond oxidation/cyclization/semipinacol rearrangement reaction; (b) tandem C–H bond oxidation/[3,3]-Cope rearrangement/aldol reaction. Figure 5: Proposed mechanism. ( a ) Tandem C–H bond oxidation/cyclization/semipinacol rearrangement reaction; ( b ) tandem C–H bond oxidation/[3,3]-Cope rearrangement/aldol reaction. Full size image Materials For NMR analysis, see Supplementary Figs 1–136 and 139–154 . For high-performance liquid chromatography traces, see Supplementary Figs 137 and 138 . For X-ray structures of the compounds, see Supplementary Figs 155–158 . General All reactions under standard conditions were monitored by thin-layer chromatography. Column chromatography was performed on silica gel (200–300 mesh). Reaction solvents were distilled before use, and all air- or moisture-sensitive reactions were conducted under an argon atmosphere. Melting points were measured using a micro-melting point apparatus. Optical rotations were measured using a 0.1-ml cell with a 1-cm path length. 1 H NMR and 13 C NMR spectra were recorded in CDCl 3 on a 400-MHz instrument ( 1 H NMR) and a 100-MHz instrument ( 13 C NMR); spectral data were reported in p.p.m. relative to trimethylsilane as the internal standard. Infrared spectra were recorded on a Fourier transform infrared spectrometer. High-resolution mass spectral analysis data were measured using the electrospray ionization technique on a Fourier transform ion cyclotron resonance mass analyser. General procedure for this tandem reaction To a solution of 1a (249 mg, 0.78 mmol) in CH 2 Cl 2 (8.0 ml), we successively added a 4-Å molecular sieve (400 mg), 2,6-DBP (924 mg, 3.90 mmol, 5.0 equiv.) and InCl 3 (18 mg, 0.08 mmol, 0.1 equiv.) at room temperature under an argon atmosphere. The mixture was stirred for 15 min, then DDQ (361 mg, 98%, 1.56 mmol, 2.0 equiv.) was added. The resulting brown mixture was stirred for 12 h at room temperature before it was filtered via an SiO 2 column with petroleum ether/EtOAc (4:1) as eluent to remove the molecular sieve and 2,6-DBP. The filtrate was concentrated under vacuum and chromatographed on an SiO 2 column (petroleum ether/EtOAc, 10:1) to give product 2a as a colourless oil (128 mg, 0.63 mmol, 81% yield). Accession codes: The X-ray crystallographic coordinates for structures reported in this study have been deposited at the Cambridge Crystallographic Data Centre (CCDC), under deposition numbers 1000817, 1000816, 1000811 and 1000827. These data can be obtained free of charge from The Cambridge Crystallographic Data Centre via www.ccdc.cam.ac.uk/data_request/cif . How to cite this article: Jiao, Z-W. et al. Tandem C–H oxidation/cyclization/rearrangement and its application to asymmetric syntheses of (−)-brussonol and (−)-przewalskine E . Nat. Commun. 6:7332 doi: 10.1038/ncomms8332 (2015).